Structure of the full-length HCV IRES in solution The 5′-untranslated region of the hepatitis C virus genome contains an internal ribosome entry site (IRES) that initiates cap-independent translation of the viral RNA. Until now, the structural characterization of the entire (IRES) remained limited to cryo-electron microscopy reconstructions of the (IRES) bound to different cellular partners. Here we report an atomic model of free full-length hepatitis C virus (IRES) refined by selection against small-angle X-ray scattering data that incorporates the known structures of different fragments. We found that an ensemble of conformers reproduces small-angle X-ray scattering data better than a single structure suggesting in combination with molecular dynamics simulations that the hepatitis C virus (IRES) is an articulated molecule made of rigid parts that move relative to each other. Principal component analysis on an ensemble of physically accessible conformers of hepatitis C virus (IRES) revealed dominant collective motions in the molecule, which may underlie the conformational changes occurring in the (IRES) molecule upon formation of the initiation complex. Hepatitis C virus (HCV) chronically infects over 170 million people worldwide and kills >350,000 people every year [1] . Its positive-strand RNA genome serves as a template for synthesis of a single precursor polypeptide that is subsequently processed by viral and cellular proteases [1] . The initiation of protein synthesis by the host–cell translation machinery occurs by a cap-independent mechanism [2] . The 5′- untranslated region of the viral RNA genome contains an internal ribosome entry site (IRES), encompassing nucleotides 39 to 371 [3] , [4] , [5] . This IRES specifically recruits the 40S ribosomal subunit to the start AUG codon without scanning [6] , [7] , [8] . Next, the IRES-40S complex interacts with the eukaryotic multi-subunit initiation factor 3 (eIF3) and the ternary Met-transfer RNA (tRNAi)-eIF2-GTP complex, forming a 48S IRES-preinitiation complex. GTP hydrolysis triggers the release of the initiation factors and the binding of the 60S ribosomal subunit, leading to the assembly of an elongation-competent IRES-80S initiation complex [9] , [10] , [11] , [12] . The IRES RNA is predicted to consist of three structural domains forming two long stem loops (domains II and III) and a spur (domain IV) ( Supplementary Fig. S1 ) [13] . The molecule contains tertiary fold motifs, the IIIabc four-way junction and the IIIef/IV pseudoknot [4] , [14] , [15] , and adopts a defined ion-dependent fold under physiological conditions [16] , although it does not form a compact, globular structure [13] , [16] , [17] . The structure at atomic resolution has been determined for several autonomous folding regions, including domain II, the III abc junction and, more recently, the III ef /IV pseudoknot [18] , [19] , [20] , [21] , [22] , [23] , [24] . The presence of several hairpin loops and regions predicted to be single-stranded likely confers dynamic flexibility to the entire IRES molecule [13] , [16] , [23] and has so far hampered structure determination of the entire molecule by X-ray crystallography or electron microscopy. As the IRES is essential for viral replication and its sequence is well conserved among all HCV genotypes, its structure represents a novel target for drug design [25] . To date, the only structural information available about the architecture of the entire IRES molecule comes from cryo-electron microscopy (cryo-EM) reconstructions of the IRES in complexes with cellular partners [26] , [27] , [28] . In these low-resolution structures, the HCV IRES adopts similar elongated conformations [26] , [27] , [28] . Upon formation of the 48S IRES-preinitiation complex, the basal part of domain III binds to the solvent-exposed side of the ribosomal 40S subunit, whereas the apical part binds to eIF3 [9] , [12] , [26] ( Supplementary Fig. S1 ). Little is known about the structure of the entire IRES in solution [13] and an atomic structure of this molecule in its free form would help to rationalize the conformational changes that occur during the assembly of the initiation complex. Characterizing the structure of large flexible macromolecules remains, however, a challenge. Recent advances in small-angle scattering of X-rays (SAXS) or neutrons have turned these methods into powerful tools for characterizing the shape and accessible conformational space of flexible macromolecules and macromolecular assemblies [29] , [30] . Combining small-angle scattering data with other structural and biophysical experimental observations or with computational approaches led to the characterization of various proteins, RNAs and multi-molecular complexes [29] . Previous biochemical studies and structural characterizations of different RNA fragments suggest that the free HCV IRES is an articulated molecule in which long structured parts are linked by flexible joints [16] , [18] , [28] . Here we built structural models of the entire isolated HCV IRES molecule and characterized its dynamics by SAXS, biomolecular simulations and computational tools. We provide experimental evidence supporting this model and found that the HCV IRES is best represented by an ensemble of conformers and identified collective motions at the origin of this conformational heterogeneity. SAXS experiments Recombinant RNA molecules corresponding to the entire IRES region of the HCV genome (nucleotides 39–371) and to four fragments were produced by in vitro transcription and purified in large amount (>10 mg) ( Supplementary Fig. S1 ). The different RNA molecules migrated as single bands on denaturing gels and behaved as monodispersed samples in dynamic light scattering experiments indicating the homogeneity of the preparations ( Supplementary Fig. S1 ). SAXS intensity was measured as a function of the scattering vector, Q. Direct analysis of these data provides additional sample quality controls and information about the degree of compactness of the particle. In the presence of 2.5 mM Mg 2+ , the Guinier plot at low Q values, in the range where Q . R g is lower than 1.5, was linear and independent of RNA concentration indicating monodisperse samples ( Fig. 1a ). Provided that concentration is known, the molecular mass of the scattering particle can be calculated from the intercept, I(0). The radius of gyration, R g , which describes the mass distribution of the particle about its centre of gravity, can be calculated from the slope. The molecular masses calculated from I(0) agree with the expected molecular masses calculated from the nucleotide sequences within experimental errors committed on concentration measurements ( Supplementary Table S1 ). 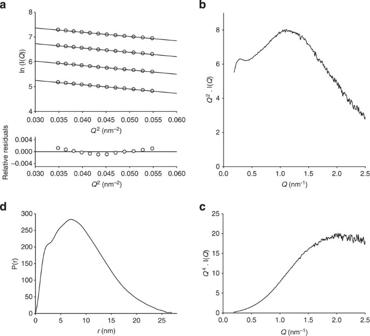Figure 1: SAXS of full-length IRES. (a) Guinier plot. Scattering curves were recorded at 1.25, 2.5, 5 and 10 mg ml−1. According to Guinier approximation, at lowQvalues, the scattering intensity of a homogeneous sample can be represented by a Gaussian function, and the Guinier plot, ln(I(Q)) as a function ofQ2, is linear. This plot is sensitive to the presence of aggregates and provides estimates for the molecular mass and the radius of gyration of the scattering particle. The lower panel shows a plot of the relative residuals obtained for a linear fit with the sample at 5 mg ml-1. Similar residual plots were obtained with the other concentrations. (b) Kratky plot. The Kratky plot (I(Q).Q2as a function ofQ) exhibits a bell shape typical of globular particles, whereas it exhibits a plateau at largeQvalues for disordered polymeric chains. (c) Porot-Debye plot. The Porod-Debye plot (I(Q).Q4as a function ofQ) tends asymptotically to a constant value as expected for compact particles, but not for flexible macromolecules. (d) Pair distances distribution function. The curve was calculated by indirect Fourier transform using the programme GNOM. Figure 1: SAXS of full-length IRES. ( a ) Guinier plot. Scattering curves were recorded at 1.25, 2.5, 5 and 10 mg ml −1 . According to Guinier approximation, at low Q values, the scattering intensity of a homogeneous sample can be represented by a Gaussian function, and the Guinier plot, ln(I( Q )) as a function of Q 2 , is linear. This plot is sensitive to the presence of aggregates and provides estimates for the molecular mass and the radius of gyration of the scattering particle. The lower panel shows a plot of the relative residuals obtained for a linear fit with the sample at 5 mg ml -1 . Similar residual plots were obtained with the other concentrations. ( b ) Kratky plot. The Kratky plot (I( Q ). Q 2 as a function of Q ) exhibits a bell shape typical of globular particles, whereas it exhibits a plateau at large Q values for disordered polymeric chains. ( c ) Porot-Debye plot. The Porod-Debye plot (I( Q ). Q 4 as a function of Q ) tends asymptotically to a constant value as expected for compact particles, but not for flexible macromolecules. ( d ) Pair distances distribution function. The curve was calculated by indirect Fourier transform using the programme GNOM. Full size image For full-length IRES, the Guinier plot at different concentration was rather linear, but the plot of the residuals showed a slight deviation from linearity ( Fig. 1a ). Deviations from linearity or concentration dependence of R g indicate aggregation or intermolecular interactions, but here the relative amplitude of the deviation is about ±0.002 ( Fig. 1a ), suggesting the absence of significant aggregation. The radius of gyration of full-length HCV IRES increased with MgCl 2 concentration, while I(0) remained constant indicating an ion-dependent conformational change and confirming the requirement of 2.5 mM Mg 2+ for proper refolding of the molecule [16] ( Supplementary Fig. S1 ). Also, in the presence of 2.5 mM MgCl 2, full-length IRES eluted as single peak on a size exclusion chromatography column and migrated as a single band on native gel indicating the absence of aggregation or of alternative folding ( Supplementary Fig. S1 ). The Kratky plot was bell shaped and the Porod-Debye plot tended asymptotically to a constant value indicating that the RNA molecule is compact particles and contain no long disordered regions ( Fig. 1b ) ( [31] , [32] , [33] ). Finally, the pair distance distribution functions, P(r), obtained by Fourier transformed of the SAXS profile, is asymmetric with maximum frequency at a distance shorter than half the maximum linear distance ( D max ) between two scattering centres, indicating that the molecules is rather elongated ( Fig. 1d ). Assembly and refinement of an atomic structure of HCV IRES In a first approach, we constructed low-resolution models of the entire IRES and of its different fragments with the programme DAMMIN [34] , [35] ( Supplementary Fig. 2 ). This programme models a macromolecule as an assembly of scattering beads arranged in space such that the calculated scattering curve reproduces the experimental curve. The shape of these optimized bead models were sufficiently irregular for allowing the docking of the known atomic structures ( Supplementary Note 1 ). In a second approach, we manually constructed an atomic model of the entire IRES that incorporates the known atomic structures (PDB accession codes 1p5o.pdb - domain II; 1kp7.pdb - domain IIIb; 1kh6.pdb - junction IIIabc; 3t4b.pdb - pseudo-knot IIIef/IV; 1f84.pdb - domain IIId, Fig. 2a ), and to refine this model, we used a multi-step procedure that generated an ensemble of 8,000 different physically realistic conformations accessible to the RNA molecule in solution. To optimize the diversity of this ensemble, we combined molecular dynamics (MD) simulations in explicit solvent (ESMD), which probes local structural fluctuations, and normal mode analysis (NMA), which explores concerted, large scale motions ( Supplementary Fig. S3 ). We then searched in this pool of conformers the unique model that minimized the discrepancy between the experimental and calculated SAXS curves. A χ -value of 10 was obtained when the calculated SAXS curve for the initial model was compared with the experimental curve, whereas a χ -value of 2.8 was obtained for the best conformer selected in the pool of 8,000 conformers ( Fig. 2b ). In this selected conformer, domains II and III extend in opposite directions along the main axis of the molecule, whereas subdomain III d and domain IV protrude on each side of the molecule ( Fig. 2c ). Along the main axis of the molecule, domain II roughly forms a right angle with domain III ( Fig. 2d ). 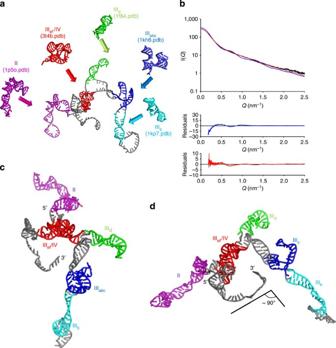Figure 2: All-atom model of HCV IRES. (a) Assembly of an all-atom model. The initial atomic model was constructed by connecting the known three-dimensional structures of the IRES fragments with single-stranded RNA or double-stranded stems in agreement with the predicted secondary structure map of theSupplementary Fig. S1. (b) Fitting the SAXS data. In the upper panel, the black curve shows the experimental SAXS curve of full-length HCV IRES, the blue curve shows the theoretical scattering curve calculated for the initial model (χ-value=10.0) and the red curve that for the refined model (χ-value=2.8). The lower panels show the plot of the residuals for the initial model and refined model, respectively. (c) and (d) Two different views of the refined model. The known three-dimensional structures of different fragments are coloured as ina. Figure 2: All-atom model of HCV IRES. ( a ) Assembly of an all-atom model. The initial atomic model was constructed by connecting the known three-dimensional structures of the IRES fragments with single-stranded RNA or double-stranded stems in agreement with the predicted secondary structure map of the Supplementary Fig. S1 . ( b ) Fitting the SAXS data. In the upper panel, the black curve shows the experimental SAXS curve of full-length HCV IRES, the blue curve shows the theoretical scattering curve calculated for the initial model ( χ -value=10.0) and the red curve that for the refined model ( χ -value=2.8). The lower panels show the plot of the residuals for the initial model and refined model, respectively. ( c ) and ( d ) Two different views of the refined model. The known three-dimensional structures of different fragments are coloured as in a . Full size image This structural model is compatible with footprint experiments preformed with chemical or enzymatic probes [16] , [36] . The accessibility of the backbone phosphorus atoms to a probe of 0.3 nm ( [37] ) is in agreement with the pattern of hydroxyl radical footprinting cleavage, predicting protections around the junction III abc and the pseudo-knot III ef /IV, but also in the internal loops of domain II ( [16] ) ( Fig. 3a ). With a larger probe (0.45 nm) that mimics the approach of a nuclease active site, the protection was predicted to be more extensive with remaining accessibility in loops II b , III a , III b and III d , as well as in domain IV, particularly at the location of the AUG codon ( Fig. 3b ). Also, as observed experimentally, the single-stranded region that connects domain II to domain III was predicted to be protected against both probes. 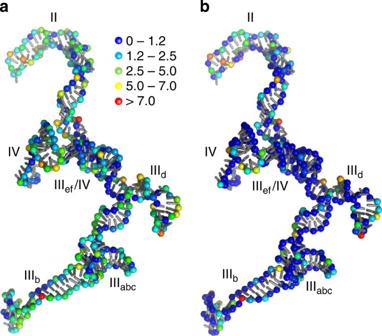Figure 3: Accessibility to the backbone phosphorus atoms. (a) Accessibilities calculated for a small probe (3.0 Å). The accessibilities were calculated with NACCESS37. The phosphorus atoms are shown as spheres and coloured according to the relative accessibility values ranging from 0 (less accessible) to >7 (most accessible) as shown in the legend. (b) Accessibility to the backbone phosphorus atoms calculated for large probe (4.5 Å). Same colour code as ina. Figure 3: Accessibility to the backbone phosphorus atoms. ( a ) Accessibilities calculated for a small probe (3.0 Å). The accessibilities were calculated with NACCESS [37] . The phosphorus atoms are shown as spheres and coloured according to the relative accessibility values ranging from 0 (less accessible) to >7 (most accessible) as shown in the legend. ( b ) Accessibility to the backbone phosphorus atoms calculated for large probe (4.5 Å). Same colour code as in a . Full size image HCV IRES is an articulated molecule in solution The HCV IRES contains two regions of tertiary fold corresponding to the four-way junction III abc and the pseudo-knot III ef /IV. Previous data suggested that the isolated four-way junction exists in a dynamic equilibrium between different conformations [38] , but ESMD simulations showed that the four-way junction is stabilized in the context of the entire domain III and that these folded elements are not major sources of flexibility in the entire IRES molecule ( Supplementary Note 2 , Supplementary Figs S4, S5 and S6 ). To localize the regions of highest flexibility in the entire IRES molecule, we ran 25 ns ESMD simulations ( Fig. 4a ) and determined the average root-mean square fluctuations over these MD trajectories ( Fig. 4b ). According to these results, the junction III abc , the stem III abc /III d stem, the pseudo-knot III ef /IV and the basal part of domain II form a rigid backbone scaffold. The apical part of domain II, subdomain III a , the apical loop of subdomain III b , subdomain III d , the hairpin loop of domain IV and the terminal single-stranded region of domain IV appear to be the most mobile parts of the structure. The single-stranded region connecting domains II and III exhibits a moderate mobility on this time scale, likely owing to an important frictional drag exerted by elongated domains II and III. 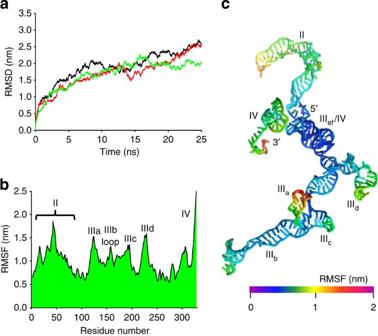Figure 4: Molecular dynamics simulation of HCV IRES. (a) Evolution of the RMSD in three independent trajectories. (b) Root-mean square fluctuations (RMSF). The RMSF values were averaged for each nucleotide over the three 20 ns MD simulations ofFig. 5a. (c) RMSF values mapped onto the model of the IRES model. The model is coloured according to the RMSF values. Figure 4: Molecular dynamics simulation of HCV IRES. ( a ) Evolution of the RMSD in three independent trajectories. ( b ) Root-mean square fluctuations (RMSF). The RMSF values were averaged for each nucleotide over the three 20 ns MD simulations of Fig. 5a . ( c ) RMSF values mapped onto the model of the IRES model. The model is coloured according to the RMSF values. Full size image Collective motions in macromolecules often dominate functional dynamics [39] . In order to identify collective motions in the IRES molecule, we applied principal component analysis to the pool of 8,000 conformations. Principal component analysis is a standard statistical method based on the analysis of covariance that is used in multiple fields for detecting correlations in large data sets. It can be used to analyse MD simulations or ensembles of conformers in order to identify collective motions of atoms in biological macromolecules [39] . Firstly, the conformers are aligned in the three-dimensional space. Secondly, covariance between atomic displacements is calculated between the different conformers, and analysing these covariance values allows identifying motions involving large numbers of atoms. Generally, a small set of collective motions, the first few principal components (PCs), capture the majority of fluctuations in biological macromolecules, and often these dominant motions have been found to be relevant for biological activities [40] , [41] . In a third step, the conformational changes corresponding to motions along each PC can be back calculated and visualized as a series of snapshots taken along the trajectories. For the 8,000 conformers of HCV IRES, the first two PCs contributed 52% of the motions within the ensemble, whereas the first six PC contributed 83% ( Fig. 5a ). The first PC corresponds to a motion of closure of the molecule, in which domains II and III remain in the same plane, acting like jaws that move towards and away from each other ( Fig. 5b ). The second component corresponds to swinging motions, in which domain II and subdomain III abc move out of their initial plane, undergoing torsions in opposite directions relative to the central pseudo-knot III ef /IV ( Fig. 5c ). The lowest and second lowest frequency modes calculated by normal mode analysis [42] corresponded to similar motions in the molecule than the first and second PC, as typically found with other biomolecules [43] . 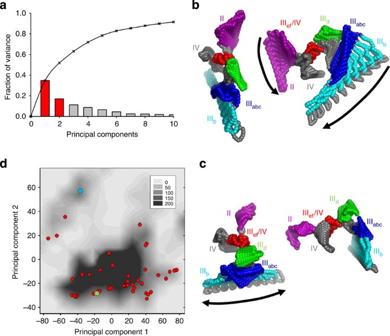Figure 5: Principal component analysis (PCA). (a) Fraction of variance (histogram) and cumulative fraction of variance (crosses) represented for the first ten PCs. PCA was applied to the ensemble of 8,000 conformers generated during the refinement process. PC1 and PC2 shown in red represent 35 and 17% of the motions. (b) Motions along the largest amplitude PC vectors. Snapshots were aken along a trajectory corresponding to the first PC, and the different conformers were superimposed by aligning their IIIef/IV pseudo-knot. The arrows indicate the direction of the main intramolecular motions. (c) Motions along the second PC. Same asFig. 5b. (d) Distribution of individual conformers along the first two PC. The grey background shows the density of population for the initial ensemble of 8,000 conformers. The green circle is for the unique model that best fitted the experimental SAXS data (shown inFig. 2c). The red circles are for models selected in ensembles of 5, 10 or 50 conformers that fit the SAXS profile. The blue circle is for the model that best matched the cryo-EM density map of the IRES bound to eIF3. Figure 5: Principal component analysis (PCA). ( a ) Fraction of variance (histogram) and cumulative fraction of variance (crosses) represented for the first ten PCs. PCA was applied to the ensemble of 8,000 conformers generated during the refinement process. PC1 and PC2 shown in red represent 35 and 17% of the motions. ( b ) Motions along the largest amplitude PC vectors. Snapshots were aken along a trajectory corresponding to the first PC, and the different conformers were superimposed by aligning their III ef /IV pseudo-knot. The arrows indicate the direction of the main intramolecular motions. ( c ) Motions along the second PC. Same as Fig. 5b . ( d ) Distribution of individual conformers along the first two PC. The grey background shows the density of population for the initial ensemble of 8,000 conformers. The green circle is for the unique model that best fitted the experimental SAXS data (shown in Fig. 2c ). The red circles are for models selected in ensembles of 5, 10 or 50 conformers that fit the SAXS profile. The blue circle is for the model that best matched the cryo-EM density map of the IRES bound to eIF3. Full size image Ensemble structure of HCV IRES On the basis of the small-angle scattering data, the entire molecule was modelled as an ensemble of conformers that accounted for the conformational diversity of the isolated IRES RNA and the coexistence of multiple exchanging conformations in solution [44] . Starting from the pool of 8,000 physically accessible conformers, we selected sub-ensembles of conformers that collectively reproduced the experimental scattering profile [44] ( Fig. 6a ). The quality of the fit between calculated and experimental scattering curves significantly improved when the number of conformers in the selected ensemble was increased from 1 model to 5 models showing that the IRES molecule is better represented by an ensemble of at least five conformers ( χ =1.9) than by a single conformer ( χ =2.8) ( Fig. 6b ). The R g value of the selected conformers spanned almost the same range (from 6.0 to 8.8 nm) than the initial pool of models ( Fig. 6c and Supplementary Fig. S7 ), suggesting that the IRES RNA samples a large conformational space in solution. Selecting ensembles of >5 conformers provided no significant improvement to the quality of the fit ( Fig. 6b ). 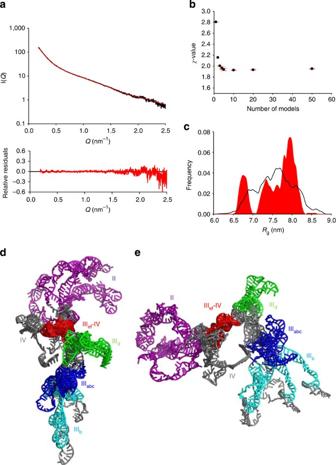Figure 6: Ensemble representation of HCV IRES. The ensemble optimization method44was used to select from the initial pool of 8,000 conformers sub-ensembles of models that collectively reproduced the experimental SAXS profile. (a) Fitting of SAXS data. The black curve shows the experimental SAXS data, and the red curve shows the theoretical curve calculated for an ensemble five conformers (χ-value=1.92). The lower graph shows the plot of the residuals. (b) Variation of theχ-value as a function of the number of conformers in the selected sub-ensemble. Theχ-values are averages of six independent selection processes. For sub-ensembles of 1–4 conformers, the same models were selected in repeated independent selections. For sub-ensembles of 5–50, different models were selected in successive selections processes and the error bars (red lines) correspond to two s.d. values of the calculatedχ-values. No difference in theχ-value was observed if the programme was allowed to select several times the same model. (c)Rgdistributions. The black curve shows the distribution ofRgin the initial pool of 8,000 conformers, whereas the red shadowed curve represents theRgdistribution for sub-ensemble of five conformers. (d) and (e) Ensemble conformation of HCV IRES. The figures show two views of one ensemble of five conformers that collectively reproduces the experimental SAXS curve as shown ina. The pseudo-knot of the five conformers was aligned, and the regions corresponding to the known atomic structures are coloured as inFig. 2. Figure 6: Ensemble representation of HCV IRES. The ensemble optimization method [44] was used to select from the initial pool of 8,000 conformers sub-ensembles of models that collectively reproduced the experimental SAXS profile. ( a ) Fitting of SAXS data. The black curve shows the experimental SAXS data, and the red curve shows the theoretical curve calculated for an ensemble five conformers ( χ -value=1.92). The lower graph shows the plot of the residuals. ( b ) Variation of the χ -value as a function of the number of conformers in the selected sub-ensemble. The χ -values are averages of six independent selection processes. For sub-ensembles of 1–4 conformers, the same models were selected in repeated independent selections. For sub-ensembles of 5–50, different models were selected in successive selections processes and the error bars (red lines) correspond to two s.d. values of the calculated χ -values. No difference in the χ -value was observed if the programme was allowed to select several times the same model. ( c ) R g distributions. The black curve shows the distribution of R g in the initial pool of 8,000 conformers, whereas the red shadowed curve represents the R g distribution for sub-ensemble of five conformers. ( d ) and ( e ) Ensemble conformation of HCV IRES. The figures show two views of one ensemble of five conformers that collectively reproduces the experimental SAXS curve as shown in a . The pseudo-knot of the five conformers was aligned, and the regions corresponding to the known atomic structures are coloured as in Fig. 2 . Full size image In order to compare the models constituting one selected ensemble, we used the programme SUPCOMB and we calculated normalized spatial discrepancy (NSD) values. The NSD parameter measure the proximity of two objects in the three-dimensional space and is analogous to the error-weighted χ -value used to characterized deviations within one-dimensional data sets [45] . Structural alignment can be performed by minimizing this parameter, and the NSD calculated between aligned structures provides a quantitative estimate of the similarity between the models. Typically, an NSD value lower than 0.7 is taken as evidence that the objects are similar. The average NSD value was always larger than 2.0, indicating that the conformers were significantly different (data not shown). Figure 6d show a representative ensemble of five models that highlights the conformational diversity of full-length HCV IRES in solution. The selected conformers of this ensemble and of other independently selected ensembles were predominantly localized in the lower part of the two-dimensional plot showing the distribution of conformers along the first and second PC for the conformational ensemble of 8,000 models ( Fig. 5d ). This suggests that motions along the first PC dominate the exchanges between the conformers of the RNA molecule in solution and that motions along the second PC are less frequent. Conformational changes in the IRES upon binding the ribosomal 40S subunit To compare the IRES structure in solution with that bound to eIF3 and the ribosomal 40S subunit, we searched within the pool of 8,000 physically accessible conformers the structure that best fitted the cryo-EM difference map ( Fig. 7 ). One model could be found for which most of domain III perfectly fitted into the cryo-EM map, but subdomain III d and domain II were not properly oriented ( Fig. 7a ). However, by applying simple rotations around two pivot points at the base of domain II and of domain III d , it was possible to slightly rearrange the IRES atomic structure such that it docked into the EM density of the bound IRES ( Fig. 7a ). The back calculated scattering curve for this conformer was significantly different from the experimental curve showing that the structure adopted by the HCV IRES in the complex with eIF3 and the 40S subunit is different from the averaged population of conformers in solution ( Supplementary Fig. S8 ). On the two-dimensional plot of PC amplitudes, the model that best matched the bound IRES is localized in the upper left corner ( Fig. 5d ), suggesting that conformational changes involving motions along the second PC mode with a reorientation of domain II relative to domain III must occur upon binding to its partners. 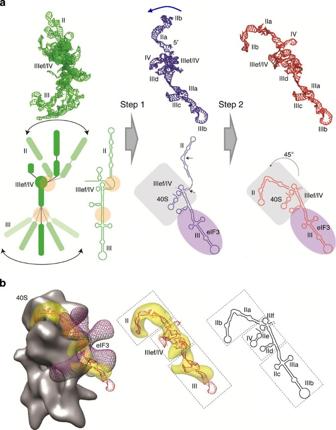Figure 7: Conformational changes upon binding to the ribosomal 40S subunit and eIF3. (a) Assembly of the IRES-preinitiation complex. HCV IRES in solution is better represented by an ensemble of conformers than by a single structure (left panel). The upper left panel shows an ensemble of five conformers that reproduce the SAXS curve. The main hinge regions, shown on both structural scheme and secondary structure map, are at the junctions of domain II with the central IIIef/IV pseudo-knot and at the base of subdomain IIIabc(orange dots in lower left panel). We propose that the assembly of the preinitiation complex starts with the binding of the basal region of IRES domain III to the back of the ribosomal 40S subunit (Step 1) followed with the binding of the apical region of IRES domain III to eIF3. The conformer from our pool of 8,000 structures that best fits into the cryo-EM reconstruction of the IRES-preinitiation complex is shown in the upper middle panel (in blue). Domain II of this conformer, clearly, did not fit into the EM reconstruction. However, by simply swivelling rigid segments of the molecule around two pivot points (arrows in the lower middle panel) it is possible to dock the atomic structure into the cryo-EM reconstruction as shown inFig. 7b, suggesting that in a second step (Step 2), domain II reorient and bind into the decoding centre of the 40S subunit (in red in th right panel). (b) HCV IRES bound to the 40S subunit and eIF3. The left panel shows the cryo-EM reconstruction of the IRES-preinitiation complex with ribosomal 40S subunit in grey, the eIF3 complex in violet and the IRES in yellow (left panel). The atomic structure docked into the cryo-EM map is shown in red. The middle panel shows the overlay of this structure with the cryo-EM difference density corresponding to the IRES extracted from the eIF3-HCV reconstruction27. The right scheme indicates the location of the different domains and subdomains of full-length IRES in its bound conformation. The dotted boxes frame the main regions of the IRES RNA, namely domain II, subdomain IIIef/IV and domain III. Figure 7: Conformational changes upon binding to the ribosomal 40S subunit and eIF3. ( a ) Assembly of the IRES-preinitiation complex. HCV IRES in solution is better represented by an ensemble of conformers than by a single structure (left panel). The upper left panel shows an ensemble of five conformers that reproduce the SAXS curve. The main hinge regions, shown on both structural scheme and secondary structure map, are at the junctions of domain II with the central III ef /IV pseudo-knot and at the base of subdomain III abc (orange dots in lower left panel). We propose that the assembly of the preinitiation complex starts with the binding of the basal region of IRES domain III to the back of the ribosomal 40S subunit (Step 1) followed with the binding of the apical region of IRES domain III to eIF3. The conformer from our pool of 8,000 structures that best fits into the cryo-EM reconstruction of the IRES-preinitiation complex is shown in the upper middle panel (in blue). Domain II of this conformer, clearly, did not fit into the EM reconstruction. However, by simply swivelling rigid segments of the molecule around two pivot points (arrows in the lower middle panel) it is possible to dock the atomic structure into the cryo-EM reconstruction as shown in Fig. 7b , suggesting that in a second step (Step 2), domain II reorient and bind into the decoding centre of the 40S subunit (in red in th right panel). ( b ) HCV IRES bound to the 40S subunit and eIF3. The left panel shows the cryo-EM reconstruction of the IRES-preinitiation complex with ribosomal 40S subunit in grey, the eIF3 complex in violet and the IRES in yellow (left panel). The atomic structure docked into the cryo-EM map is shown in red. The middle panel shows the overlay of this structure with the cryo-EM difference density corresponding to the IRES extracted from the eIF3-HCV reconstruction [27] . The right scheme indicates the location of the different domains and subdomains of full-length IRES in its bound conformation. The dotted boxes frame the main regions of the IRES RNA, namely domain II, subdomain III ef /IV and domain III. Full size image On the basis of SAXS experiments, we built bead models, as well as unique and ensemble atomic models in which the IRES RNA appears to be non-globular. Domain II and domain III form independent long cylindrical stems that extend in different directions from the central III ef /IV pseudo-knot and constitute the dorsal spine of a structure from which subdomains III a , III c and III d and domain IV protrude on the sides. This structural architecture is in agreement with electron microscopy pictures of free HCV IRES [13] . In addition, the atomic model is in agreement with available biochemical data, in particular, with experimental accessibilities measured for chemical and enzymatic probes [16] . A comparison of the different modelling approaches highlights the dynamic character of the molecule. Ensemble structures of five or more conformers provide better fits to the experimental data than a single atomic structure suggesting a static or dynamic heterogeneity of the structure, and raising the question of why an ensemble of five conformers is necessary and sufficient to reproduce the experimental curve. Our results argue against static heterogeneity in solution. Indeed, different ensembles of conformers can reproduce the experimental data as well, and if large ensembles were selected no conformer was statistically overrepresented in the population. The small size of the ensemble required for reproducing the scattering curve more likely results from the low information content of SAXS data, reporting only on the pair distance distribution between scattering centres. Because of this low structural resolution, an ensemble of five conformers is sufficient for representing the conformational diversity of a molecule that is continuously sampling an enormous number of conformations under thermal motions [44] ( Fig. 7a ). In consequence, the conformers of one peculiar selected ensemble should not be taken as actual structures of free HCV IRES, but rather as mere examples of structures that collectively represent the molecule in solution. Molecular dynamics simulations, principal component analysis and ensemble modelling of SAXS data reveal motions in the RNA molecules that may potentially be relevant to the rearrangement of the IRES molecule occurring during the assembly of the 48S preinitiation complex and initiation complex [46] , [47] . The selected models that represent the IRES in solution have values of the first component distributed along the entire range sampled in the initial ensemble, whereas they have values of the second component falling in a more limited range of the initial ensemble ( Fig. 5d ). This suggests that the isolated IRES molecule undergoes motions that mainly correspond to the first PC. Upon binding to its cellular partners, the conformational flexibility of the IRES seems to be significantly reduced leading to the visualization of the molecule in the cryo-EM reconstructions of the different complexes, although the shape and width of the electron density suggest that the IRES RNA conserves some flexibility in its bound state [27] , [28] ( Fig. 7c ). principal component analysis suggests that the conversion of the conformers most frequently present in solution into the bound conformer requires motions through the second PC ( Fig. 7a ). Two limiting mechanisms, conformational selection or conformational change after binding, can be considered for the assembly of the flexible IRES molecule with its partners during the formation of the initiation complex. In the first mechanism, only IRES molecules adopting the bound conformation in solution can bind to their partners. As the bound conformation is accessible to the molecule in solution through its main concerted motions, there is an inherent probability that IRES will adopt this conformation and, therefore, bind to its partners. The bound conformer appears to be lowly populated in solution ( Fig. 5d ), however, it should be noted that our structural characterization of HCV IRES was carried out in dilute solutions. It is possible that the complex cellular environment affects the conformational properties of the molecule and enhances the population of preorganized conformers capable of binding. In the second mechanism, various conformers of the IRES would bind to the partners and would then undergo conformational changes to adapt their shape to the binding site. It is difficult to distinguish between these two scenarios [48] , and there is always the possibility that a combination of both mechanisms is involved in the recruitment of the 40S ribosomal subunit and of eIF3 by HCV IRES. As domains II and IV are required for efficient translation in vitro and in vivo [7] , [26] , [36] but provide no significant stabilization to the IRES-preinitation complex [7] , [9] , [12] and that domain III has a slightly higher affinity for the ribosomal 40S subunit than for eIF3 [7] , [12] , it is tempting to speculate that domain III binds first onto the back of the ribosomal 40S subunit, and subsequently to eIF3, and that conformational changes occur in the complex ( Fig. 7a ). In particular, motions along the second PC may take place in order to correctly position domain II within the tRNA exit (E) site and the mRNA binding cleft of the ribosome and to trigger conformational changes in the 40S subunit and in the IRES [26] , [28] , [46] , [47] ( Fig. 7a ). This would commit the complex to progress towards the conformational reorganization of domain IV that contains the start AUG codon and the correct positioning of this domain into the ribosome decoding centre [12] . The concerted motions of the IRES revealed in this study, in particular those according to the second PC, could explain this long range communication within the IRES molecule. Conformational dynamics thus appears as an inherent property of the HCV IRES molecule that may be biologically relevant. The IRES sequence is highly conserved among the genotypes of HCV, and the localization of the variations in our structural model suggests that the dynamics of the molecule is conserved among the different genotypes. Indeed, variations in loops unlikely affect the dynamics and variations in stem regions are always complemented such that base pairing is conserved. IRES have been found in the RNA genomes of different viruses and in some cellular mRNA [49] . They have been divided in four groups on the basis of their predicted secondary structure and on their requirements for initiation factors and other cellular factors [50] . A common feature of all IRES is their inherent flexibility, which seems to increase in correlation with the need for more initiation factors. HCV IRES belongs to class II IRES and requires eIF3, eIF2 and initiator met-tRNA to assemble ribosomes [10] . We showed here that it is an articulated molecule in which structured elements undergo large reorientations relative to each other [16] , [18] , [28] . By comparison, IRES of group I found in the intergenic region of Dicistroviridae assemble ribosome in the absence of canonical initiation factors and Met-tRNA and undergo only local rearrangements upon formation of the initiation complex [51] , [52] , [53] . The structure of group I IRES is composed of two well-structured regions for which atomic structures have been obtained [54] , [55] . Groups III and IV, which require most of the canonical initiation factors, as well as some IRES trans-acting factors for assembling ribosome, exhibit no protection against enzymatic or chemical probes in their free form suggesting that they are more dynamics than HCV IRES [50] . Only IRES of groups I and II bind directly to the 40S ribosomal subunit, whereas IRES of groups III and IV interact with the ribosomal subunits only in the form of ribonucleoprotein complexes, and currently, structural data are only available for groups I and II IRES. Despite their differences in structural architecture and dynamics, IRES of groups I and II share similarities in the way they recruit and manipulate ribosomal subunits. The structure of the IRES of both classes is grossly composed of two parts that have similar functions in ribosome assembly. A first part is responsible for tight binding to the ribosomal 40S subunit, although the binding site is localized in different regions of the 40S subunit. Domain II of intergenic region IRES binds to the evolutionary conserved region of the 40S subunit that interacts with the 60S subunit, whereas domain III of HCV binds to the less conserved solvent-exposed backside of the 40S subunit. The second part tinkers with the decoding centre of the ribosome but provides no additional stabilization to the complex with the 40S subunit. Domain III of the intergenic region IRES mimics tRNA in a hybrid state [54] and binds to the A site, whereas domain II of HCV IRES binds close to the E site and domain IV inserts into the P site [47] . In conclusion, both intergenic region IRES and HCV IRES alter the conformation of the 40S subunit upon binding and change of conformation upon binding the 60S subunit. The inherent flexibility of HCV IRES as highlighted in this study may thus have an important role in the assembly and manipulation of the ribosomal subunits and, in the case of HCV, may be controlled by the binding of the initiation factors. RNA synthesis by in vitro transcription cDNA (HCV genotype 1b – NCBI nucleotide accession number AJ238799) corresponding to the different constructs were amplified by PCR. The forward oligonucleotide included an Eco RI site and the T7 RNA polymerase promoter followed by a triple G sequence in order to increase transcriptional activity, and the reverse oligonucleotide included a Hin dIII site. Each fragment was cloned into pUC18 between the Eco RI and Hin dIII restriction sites. RNA corresponding to HCV IRES and its different fragments were prepared by in vitro transcription from linearized plasmids using T7 RNA polymerase as described in Supplementary methods online . Samples for SAXS experiments were prepared by dissolving 1 mg of RNA in 50 μl of water and incubating the solution for 10 min at room temperature without shaking. Samples were heated for 3 min at 95 °C and incubated for 5 min at room temperature before adding 50 μl of refolding buffer (40 mM Tris–HCl buffer at pH 7.5 containing 200 mM KOAc, 400 mM KCl, 5 mM MgCl 2 and 1 mM dithiothreitol). The samples were then incubated for 10 min at room temperature. Concentration was measured by absorbance at 260 nm and was adjusted to 10 mg ml −1 . Small-angle X-ray scattering experiments SAXS data were collected at the European Synchrotron Radiation Facility (Grenoble, France) on beamlines ID2 and ID14-3 (see the Supplementary methods online for additional details). Generation of an atomic model of the full-length HCV IRES An initial atomic model of HCV IRES was reconstructed by using base pairing information from the secondary structure map and the known atomic structures of fragments. The non-natural nucleotides present in some atomic structures were replaced by natural nucleotides. The regions of unknown structure were constructed with COOT [56] as stems or loops in accordance with the secondary structure map. The different fragments were progressively assembled; one by one they were correctly positioned in space using the bead model of full-length IRES as a guide and they were connected in VEGA ZZ [57] . After the assembly of each fragment, local energy minimization was performed in VEGA ZZ to remove potential interatomic clashes between the pre-existing and newly added parts of the structure [57] . The model of the entire IRES was globally energy-minimized in GROMACS using the AMBER99 force field. This model was then refined by a multiple step protocol, described below, that combines ESMD and NMA to identify a model that minimize the discrepancy between the experimental and calculated scattering curve using the χ -value: where K is the number of points in the experimental curve, σ is the s.d. and μ is a scaling factor. Explicit solvent molecular dynamics simulations All molecular dynamics simulations were performed with the GROMACS 4 software package using different force fields. For the equilibration process and production runs used for refining the model, we used an ensemble of harmonic restraints between the 63 GC base pairs present in the initial model in order to enforce native local secondary structure. The system was equilibrated for 250 ps or 1 ns, and we verified that both potential and kinetic energies had reached equilibrium at the end of this equilibration. Independent production simulations with or without harmonic restraints were obtained by using different initial velocities. The resulting trajectories were analysed using GROMACS routines to extract root mean square deviation (RMSD), root-mean square fluctuations and R g information (see Supplementary methods online for details and references). Structure refinement Starting from the manually assembled structure, an ensemble of models was generated by a multi-step procedure in which we combined ESMD, NMA and molecular modelling ( Supplementary Fig. S3 ). In a first step, starting from the energy-minimized all-atom model, we ran six independent ~20 ns ESMD simulations with the 63 harmonic restraints using the AMBER99 force field. In each MD trajectory, after a rapid rise in the first 2 ns, the RMSD evolved towards a stable value near 2.5 nm and the R g value decreases. Two-thousand four-hundred conformers were obtained as snapshots taken at regular interval (50 ps) along the six first MD simulations, and the theoretical scattering profiles were calculated from the structures using the programme CRYSOL [58] and compared with the experimental data. The best agreement with the experimental curve yielded a χ -value of 6, down from a value of 10 calculated for the initial structure. A summary of the conformational sampling performed during this first refinement step is shown in the form of plots of R g versus χ -value ( Supplementary Fig. S3 ). In a second step, in order to expand the sampled conformational space, the best fitting model of each MD simulation was submitted to normal mode calculation (NMA) using the elNémo web-server [42] . For each of these 6 models, 40 structures were extracted (using an amplitude of motion equal to ±1000 and a step of 50) from each of the five lowest frequency normal modes, yielding 1,200 additional models ( Supplementary Fig. S3 ). The theoretical scattering profiles were compared with the experimental profile. The best agreement with the experimental profile yielded a χ -value of 4.3. To further increase the conformational sampling, the best model selected after NMA was energy-minimized and submitted to four additional ~20 ns ESMD simulations using AMBER99 and the harmonic restraints ( Supplementary Fig. S3 ). One-thousand six-hundred additional conformers were obtained by taking at regular interval (50 ps) along these trajectories and the calculated scattering profile was compared with the experimental data, but no improvement in the fitting was obtained with these models (best agreement yielded a χ -value of 4.0). Finally, we noticed that reorientations of domain II relative to domain III occurred during the ESMD simulations, but that this type of concerted motion was slow and was thus infrequent on the simulated timescale. To improve the conformation sampling generated by this motion, starting from the best model selected after the last four ESMD with AMBER99, we used the elNémo web-server [42] with a large amplitude of motion (±2,000) and selected five snapshots from the lowest frequency mode of motion (4 × 5=20 models). These models were energy-minimized in GROMACS and were used to generate additional models by randomly rotating domain II around a pivot point located in a single-stranded region at the intersection between domains II and III (nucleotides 119–124). For each of the 20 energy-minimized models, 140 models were generated with the torsion-based random conformational search functionality of Another Molecular Mechanics Program (AMMP) implemented in VEGA ZZ, leading to 2,800 additional conformers. A model with a χ -value of 2.8 between the experimental and calculated curve was finally selected using CRYSOL [58] ( Fig. 2 ). Six additional ~25 ns ESMD simulations using AMBER99 parmbsc0 were run with or without applying harmonic restraints on the 63 GC base pairs. Three-thousand additional conformers were obtained by taking snapshots at regular interval (50 ps) along these trajectories and their calculated scattering profiles were compared with the experimental data, but no improvement in the fitting was obtained with these models. Although, no major difference was found between the trajectories calculated with the two force fields, only the three trajectories calculated without restraints were used to calculate the root-mean square fluctuations values. Ensemble optimization All models generated during the refinement process were pooled into an ensemble of 8,000 models. This pool was used for selecting sub-ensemble that collectively reproduce the SAXS profile using the genetic algorithm GAJOE from ensemble optimization method [59] . The size of the selected ensemble was varied from 1 to 50 models in order to test the effect of the size of the ensemble on the quality of the fit. The number of generation of the genetic algorithm was adjusted to optimize the χ-value. Models of the optimized ensembles were aligned using the pseudo-knot domain as a reference using GROMACS routines. The quality of the structures constituting the selected ensembles was checked with the MolProbity webserver [60] . The pdb files of the five conformers forming the ensemble presented in Fig. 6 are available as Supplementary Data 1 . How to cite this article: Pérard, J. et al . Structure of the full-length HCV IRES in solution. Nat. Commun. 4:1612 doi: 10.1038/ncomms2611 (2012).